Reciprocal inhibition between sensory ASH and ASI neurons modulates nociception and avoidance inCaenorhabditis elegans Sensory modulation is essential for animal sensations, behaviours and survival. Peripheral modulations of nociceptive sensations and aversive behaviours are poorly understood. Here we identify a biased cross-inhibitory neural circuit between ASH and ASI sensory neurons. This inhibition is essential to drive normal adaptive avoidance of a CuSO 4 (Cu 2+ ) challenge in Caenorhabditis elegans . In the circuit, ASHs respond to Cu 2+ robustly and suppress ASIs via electro-synaptically exciting octopaminergic RIC interneurons, which release octopamine (OA), and neuroendocrinally inhibit ASI by acting on the SER-3 receptor. In addition, ASIs sense Cu 2+ and permit a rapid onset of Cu 2+ -evoked responses in Cu 2+ -sensitive ADF neurons via neuropeptides possibly, to inhibit ASHs. ADFs function as interneurons to mediate ASI inhibition of ASHs by releasing serotonin (5-HT) that binds with the SER-5 receptor on ASHs. This elaborate modulation among sensory neurons via reciprocal inhibition fine-tunes the nociception and avoidance behaviour. Sensory neurons transform various stimuli from the external and internal environment into sensory information that is primarily integrated in the central nervous system to form sensation and perception, drive adaptive behaviours and maintain physiological homeostasis. The sensory modulations at the level of sensory neurons or the initial chain of sensory pathways are important for animals to achieve direct, fast and more fine-tuned regulation of sensations and behaviours [1] , [2] , [3] . Owing to feasible genetic manipulation, a simple and stereotyped nervous system, the nematode Caenorhabditis elegans is a good animal model for the study of peripheral modulation of sensations. In C. elegans , nociceptive sensations and avoidance have been intensively studied. However, the reported studies were focused on the functional mapping of the connections among sensory neurons and interneurons, using cell ablation, optogenetic manipulation and in vivo calcium imaging [4] , [5] , [6] , [7] . Therefore, the peripheral modulation of nociceptive sensations and avoidance behaviours is poorly understood. The polymodal ASH sensory neurons in C. elegans sense a variety of aversive stimuli and mediate avoidance of high osmotic, mechanical and chemical stimuli [8] , [9] , [10] , [11] . Notably, the neurotransmitters, such as neuropeptides, serotonin (5-HT), tyramine (TA) and octopamine (OA), have been increasingly shown to be transmitters or modulators of ASH-mediated aversive behaviours [12] , [13] , [14] , [15] . ASI sensory neurons are reported to mediate dauer formation [16] , enable worms to learn to avoid the smell of pathogenic bacteria after ingestion via INS-6 signalling [17] , suppress male-specific sexual attraction behaviour [18] , respond to temperature stimuli to negatively modulate thermotaxis behaviour [19] , mediate diet-restriction-induced longevity [20] , modulate satiety quiescence [21] , regulate acute CO 2 avoidance [22] , repress exploratory behaviours that comprise spontaneous reversals and omega turns [5] , and inhibit ASH-mediated aversive responses to 100% 1-octanol [23] . These studies support the hypothesis that ASIs are important polymodal sensory neurons mediating or modulating worm behaviours and development. Here, using a reverse genetic screen as well as genetic manipulation, quantitative behaviour assays, in vivo Ca 2+ imaging and neuronal manipulation, we determine that reciprocal inhibition between ASHs and ASIs exists following a challenge of nociceptive Cu 2+ stimulation and identify the underlying molecular mechanism and neural circuit. The elaborate modulation of Cu 2+ sensation through the reciprocal inhibitory neuron circuit fine-tunes the worm nociception and avoidance behaviour. Blocking ASH and ASI alters kinematics of CuSO 4 reversal A wild-type C. elegans worm exhibits a rapid backward movement when its nose encounters water-soluble repellents in a dry drop test [24] . To quantify the kinematics of worm undulatory locomotion during a CuSO 4 -evoked reversal, we calculated the normalized curvature (NC) of the worm body [25] , [26] . In brief, the worm body was divided into ten equal segments from head to tail (head=0 and tail=1). The NC of each point along the body centre line was defined as the total length of the body centre line ( L ) divided by the radius of curvature ( R ) of the point ( Fig. 1a ). Typically, as the absolute value of the NC increases, the bending magnitude increases. We used a quadrant assay with some modifications [27] , to test the sensitivity of mass worms to CuSO 4 ( Fig. 1b ). Whereas a wild-type worm exhibited no obvious response to M13 buffer in the dry drop test ( Supplementary Movie 1 ), it generated a continuous and rhythmic sinusoidal backward locomotion when challenged with 10 mM CuSO 4 -M13 buffer solution ( Fig. 1c1 and Supplementary Movie 2 ). The bending magnitude of the reversal in the tail was stronger than that in the head ( Fig. 1d1 ), which was different from previously reported forward locomotion [26] . 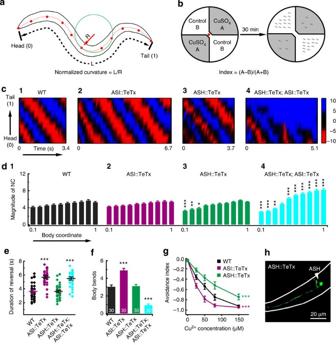Figure 1: Sensory neurons ASHs and ASIs direct the Cu2+-evoked avoidance behaviour. (a) Schematic representation of quantification of NC along the body centre line. The length of body centre lineLis divided into 10 equal segments from head (0) to tail (1) using 11 points. The radius of curvatureRat the middle point of a segment is defined as the curvature of this segment. The non-dimensional NC was calculated by dividing theLbyR. (b) Schematic representation of a modified quadrant assay. The red dot represents the starting point of the worms. (c1–c4) Kymograms of the time-dependent NC along the body centre line of Cu2+-evoked reversals in the worms after blocking different neurons by neuron-specific expression of TeTx. The data are expressed as means,n=30 assays. The vertical axis represents the midline of body from head (0) to tail (1) in non-dimensional units, and the horizontal axis represents the duration of the reversal. (d1–d4) The magnitude of body bend described inc1–c4. NC indicates normalized curvature and similarly hereinafter;n=30 assays. The durations (e) and body bends (f) of the Cu2+-elicited reversal assayed by the dry drop test in the worms after blocking neurotransmission in different neurons. The number on each bar indicates the number of independent tests for each genotype. (g) The worm avoidance indexes in response to various concentrations of Cu2+tested by the quadrant assay, that is, Cu2+sensitivity,n≥8 assays. (h) The specific expression of TeTx light chain in ASHs using a FLP–FRT site-specific recombination system. Scale bar, 20 μm. The data except those incare expressed as means±s.e.m. Two-way analysis of variance (ANOVA) test ind1–d4andg, and one-way ANOVA test ine,f. Corrected with Bonferronit-test for multiple comparisons (*P≤0.05, **P≤0.01 and ***P≤0.001 compared with the wild-type N2 control). Figure 1: Sensory neurons ASHs and ASIs direct the Cu 2+ -evoked avoidance behaviour. ( a ) Schematic representation of quantification of NC along the body centre line. The length of body centre line L is divided into 10 equal segments from head (0) to tail (1) using 11 points. The radius of curvature R at the middle point of a segment is defined as the curvature of this segment. The non-dimensional NC was calculated by dividing the L by R . ( b ) Schematic representation of a modified quadrant assay. The red dot represents the starting point of the worms. ( c1 – c4 ) Kymograms of the time-dependent NC along the body centre line of Cu 2+ -evoked reversals in the worms after blocking different neurons by neuron-specific expression of TeTx. The data are expressed as means, n =30 assays. The vertical axis represents the midline of body from head (0) to tail (1) in non-dimensional units, and the horizontal axis represents the duration of the reversal. ( d1 – d4 ) The magnitude of body bend described in c1 – c4 . NC indicates normalized curvature and similarly hereinafter; n =30 assays. The durations ( e ) and body bends ( f ) of the Cu 2+ -elicited reversal assayed by the dry drop test in the worms after blocking neurotransmission in different neurons. The number on each bar indicates the number of independent tests for each genotype. ( g ) The worm avoidance indexes in response to various concentrations of Cu 2+ tested by the quadrant assay, that is, Cu 2+ sensitivity, n ≥8 assays. ( h ) The specific expression of TeTx light chain in ASHs using a FLP–FRT site-specific recombination system. Scale bar, 20 μm. The data except those in c are expressed as means±s.e.m. Two-way analysis of variance (ANOVA) test in d1 – d4 and g , and one-way ANOVA test in e , f . Corrected with Bonferroni t -test for multiple comparisons (* P ≤0.05, ** P ≤0.01 and *** P ≤0.001 compared with the wild-type N2 control). Full size image To identify the functions of ASI and ASH neurons in the Cu 2+ -evoked avoidance behaviour, we used the light chain of tetanus toxin (TeTx) to block ASI and ASH neurotransmission (silence or block neurons for short) [28] . TeTx is a specific protease of synaptobrevin and has been used successfully to inhibit chemical synaptic transmission in C. elegans [29] . We examined the impact of silencing ASIs on the kinematics of a Cu 2+ -evoked reversal. We observed a marked increase in the duration and body bends of the backward movements ( Fig. 1c2 and Supplementary Movie 3 ), but no change in the bending magnitude ( Fig. 1d2 ) compared with those observed in wild-type animals. We next examined the changes in the sensitivity of mass worms to Cu 2+ stimulations using the quadrant assay. Our result showed that worms displayed hypersensitivity after permanently blocking ASI neurotransmission with TeTx ( Fig. 1g ). We then explored the effects of blocking ASHs on the reversal kinematics. No ASH-specific promoter has been identified; therefore, we used a flippase (FLP)-flippase recognition target (FRT) site-specific recombination system to drive specific expression of TeTx in ASH neurons [29] , [30] . When worms expressed both sra-6p::flp-sl2-flp::3′UTR and gpa-11p::frt-stop-frt::TeTx::sl2-GFP constructs, FLP recombinase driven by the sra-6 promoter excised the FRT-flanked transcriptional terminator. This allowed specific expression of TeTx and a green fluorescent protein (GFP) fluorescence marker in ASH neurons that possess a combinatorial intersection between sra-6 and gpa-11 promoters [30] ( Fig. 1h ). Specifically silencing ASH neurons significantly decreased the bending magnitude of the worm anterior body region ( Fig. 1c3 and Supplementary Movie 4 ), had no impact on the duration and the body bend of the reversal ( Fig. 1e,f ), and also significantly decreased the sensitivity to Cu 2+ of the mass worms measured by the quadrant assay ( Fig. 1g ). These results demonstrated that ASHs are nociceptive Cu 2+ sensory neurons and play an important role in anterior body bending as part of the Cu 2+ avoidance behaviour. Interestingly, blocking both ASH and ASI neurons induced a serious uncoordinated reversal and even irreversible backward locomotion. Only bends of weak magnitude remained in the anterior parts of the body ( Fig. 1c4 and Supplementary Movie 5 ). ASIs inhibit ASHs to regulate worm aversive behaviour As blocking ASI affects worm aversive behaviour and sensitivity to Cu 2+ , we next addressed the underlying mechanism. We first monitored Ca 2+ transients in ASHs using the genetically encoded Ca 2+ sensor R-GECO1 ( Fig. 2a ), which has properties of high Ca 2+ affinity, a large dynamic range and slow photobleaching [31] . A transparent polydimethylsiloxane microfluidic device was used to trap and expose worms to the Cu 2+ stimulus [32] , [33] . ASHs showed an obvious on- and off-response that precisely corresponded to the presentation and removal of the noxious stimulus, respectively, following a 30-s stimulation with 10 mM CuSO 4 ( Fig. 2b , Supplementary Fig. 1 and Supplementary Movie 6 ). However, ASIs showed only an off-response of Ca 2+ transient but no apparent on-response ( Fig. 2c and Supplementary Movie 7 ). We employed TeTx to permanently block ASI neurotransmission, and ArchT, a light-driven outward proton pump with high light sensitivity [34] , to optogenetically inhibit ASI neurons. Genetically silencing and optogenetically inhibiting ASIs ( Fig. 2c ) significantly prolonged the on-response of Cu 2+ -elicited Ca 2+ signals in ASH neurons ( Fig. 2b and Supplementary Movie 8 ). As expected, the optogenetic inhibition, but not the genetic blocking, markedly decreased ASI off-response Ca 2+ signals, suggesting that TeTx blocked neurotransmission but did not change ASI excitation ( Fig. 2c ). 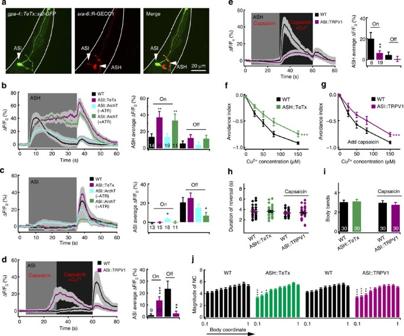Figure 2: ASIs inhibit ASH Cu2+-elicited Ca2+response and worm avoidance. (a) Expression of TeTx in ASIs and R-GECO1 in ASHs. Scale bar, 20 μm. ASH (b) and ASI (c) Ca2+responses to a 10-mM Cu2+stimulation after blocking or during optogenetic inhibition of neurotransmission in ASIs. ‘On’ and ‘Off’ indicate Ca2+signals to the presentation and removal of the Cu2+stimulation, respectively. For calculating the ratio of ΔF/F0, the ΔFandF0for the on-response are defined as the fluorescence changes during the application of CuSO4and the average fluorescence intensity of 5 s before the Cu2+stimulation, and the ΔFandF0for off-response are defined as the initial fluorescence changes 5 s after the removal of CuSO4and the average fluorescence intensity of the last 5 s of the on-response, respectively. Grey shading denotes the period of Cu2+application. For ArchT optogenetic inhibition, continuous green light irradiation was applied during the entire recording, ATR, all-trans-retinal; similarly herein after. The ASI (d) and ASH (e) Ca2+signals in response to the 10 mM CuSO4stimulation following chemogenetic activation of ASIs. Neurons that specifically expressed TRPV1 were activated by exogenous capsaicin (100 μM). TheF0of the on-response was defined as the average fluorescence intensity from 0 to 5 s. Light grey and dark grey shading denote the span of applications of capsaicin and capsaicin plus Cu2+, respectively; similarly herein after. Comparison of Cu2+sensitivity tested by the quadrant assay (f,g,n≥8 assays) and kinematics of the Cu2+-evoked reversal in the dry drop test (h–j,n=30 assays) after genetically blocking ASHs with TeTx or chemogenetically exciting ASIs with TRPV1 plus 10 μM capsaicin. All data are expressed as means±s.e.m. The number on each bar indicates the number of independent tests for each genotype. One-way analysis of variance (ANOVA) test inb–eandh,i, and two-way ANOVA test inf,g,j. Corrected with Bonferronit-test. Statistical significance was indicated as: *P≤0.05, **P≤0.01 and ***P≤0.001. Figure 2: ASIs inhibit ASH Cu 2+ -elicited Ca 2+ response and worm avoidance. ( a ) Expression of TeTx in ASIs and R-GECO1 in ASHs. Scale bar, 20 μm. ASH ( b ) and ASI ( c ) Ca 2+ responses to a 10-mM Cu 2+ stimulation after blocking or during optogenetic inhibition of neurotransmission in ASIs. ‘On’ and ‘Off’ indicate Ca 2+ signals to the presentation and removal of the Cu 2+ stimulation, respectively. For calculating the ratio of Δ F / F 0 , the Δ F and F 0 for the on-response are defined as the fluorescence changes during the application of CuSO 4 and the average fluorescence intensity of 5 s before the Cu 2+ stimulation, and the Δ F and F 0 for off-response are defined as the initial fluorescence changes 5 s after the removal of CuSO 4 and the average fluorescence intensity of the last 5 s of the on-response, respectively. Grey shading denotes the period of Cu 2+ application. For ArchT optogenetic inhibition, continuous green light irradiation was applied during the entire recording, ATR, all-trans-retinal; similarly herein after. The ASI ( d ) and ASH ( e ) Ca 2+ signals in response to the 10 mM CuSO 4 stimulation following chemogenetic activation of ASIs. Neurons that specifically expressed TRPV1 were activated by exogenous capsaicin (100 μM). The F 0 of the on-response was defined as the average fluorescence intensity from 0 to 5 s. Light grey and dark grey shading denote the span of applications of capsaicin and capsaicin plus Cu 2+ , respectively; similarly herein after. Comparison of Cu 2+ sensitivity tested by the quadrant assay ( f , g , n ≥8 assays) and kinematics of the Cu 2+ -evoked reversal in the dry drop test ( h – j , n =30 assays) after genetically blocking ASHs with TeTx or chemogenetically exciting ASIs with TRPV1 plus 10 μM capsaicin. All data are expressed as means±s.e.m. The number on each bar indicates the number of independent tests for each genotype. One-way analysis of variance (ANOVA) test in b – e and h , i , and two-way ANOVA test in f , g , j . Corrected with Bonferroni t -test. Statistical significance was indicated as: * P ≤0.05, ** P ≤0.01 and *** P ≤0.001. Full size image We next examined the effect of activating ASIs on ASH Cu 2+ -evoked Ca 2+ signals. Worms display phototaxis [35] . Thus, to avoid the possible interference from light used in optogenetics, we employed chemical genetics using transient receptor potential vanilloid 1 (TRPV1), a mammalian cation channel activated by an exogenous ligand capsaicin, to chemogenetically activate ASI neurons [36] . Our results showed that the expression of rat TRPV1 endowed ASIs with the ability to respond to the application of 100 μM capsaicin ( Fig. 2d ). The chemogenetic activation of ASIs significantly decreased the ASH Ca 2+ transients in response to the Cu 2+ challenge ( Fig. 2e ). Moreover, artificially activating ASIs induced the identical changes in Cu 2+ sensitivity ( Fig. 2f,g ), no changes in the duration of reversal and body bend ( Fig. 2h,i ), and similar but more severe changes in the bending magnitudes in the anterior parts of the body ( Fig. 2j ) compared with blocking ASH neurons. Taken together, these results demonstrate that ASIs inhibit the ASH response to Cu 2+ and regulate the worm Cu 2+ avoidance behaviour. 5-HT mediates ASI inhibition on ASHs via the SER-5 receptor ASIs are presynaptic to ASHs ( www.wormweb.org ). For identifying ASI neural signalling, we used reverse genetics to screen neuropeptide and neurotransmitter receptors, using a standard that Cu 2+ -evoked Ca 2+ signals of ASHs were similar to those in ASI-blocked worms ( Supplementary Fig. 2 ). We found that the ser-5 loss-of-function (lof) mutations ( ser-5 ( ok3087 ) and ser-5 ( tm2647 )) had similar impacts to permanently silencing ASIs on ASH Cu 2+ -elicited Ca 2+ signals ( Fig. 3a and Supplementary Fig. 2 ), the kinematics of Cu 2+ -evoked reversal ( Fig. 3b,c ) and Cu 2+ sensitivity ( Fig. 3d ), and these mutations also had no effect on the bending magnitudes ( Supplementary Fig. 3a ). All defects in the mutants were rescued by the ectoexpression of ser-5 genomic DNA driven by its own or ASH-specific promoter in ser-5 ( ok3087 ) ( Fig. 3a–d and Supplementary Fig. 3a ). Genetically blocking ASIs and the ser-5 lof mutation had no impact on ASI Cu 2+ -elicited Ca 2+ signals as expected ( Supplementary Fig. 3b ). These data suggested that SER-5 directly mediated ASI inhibition of the ASH Cu 2+ response and thus worm aversive behaviour. ser-5 encodes a 5-HT receptor, which is widely expressed in head neurons including ASHs [37] ( Fig. 3e ). We then tested whether blocking the biosynthesis of 5-HT causes phenotypes similar to the lof mutation of ser-5. The gene tph-1 encodes tryptophan hydroxylase that catalyses the rate-limiting first step in 5-HT biosynthesis [38] . In the C. elegans hermaphrodite, tph-1 expression is limited to only a few serotonergic neurons, such as NSMs, ADFs and HSNs, and rarely in AIMs and RIH ( Supplementary Fig. 3c ). Indeed, in tph-1 ( mg280 ) mutants, which fail to synthesize 5-HT, the ASH calcium transients and the avoidance behaviours were similar to those in the ser-5 -null mutants ( Fig. 3f,h–j and Supplementary Fig. 3d ). The defects were rescued by the expression of tph-1 directed by its own promoter or the application of 5 mM exogenous 5-HT ( Fig. 3f–j and Supplementary Fig. 3d ). These results suggest that endogenous 5-HT mediates ASI inhibition of ASH neurons. Taken together, our results suggest that endogenous 5-HT directly acts on the SER-5 receptor to mediate the ASI inhibition of ASHs. However, as ASIs are not known to be serotonergic neurons, exactly which neurons release the 5-HT that regulates the ASH response and worm avoidance behaviour needs further investigation. 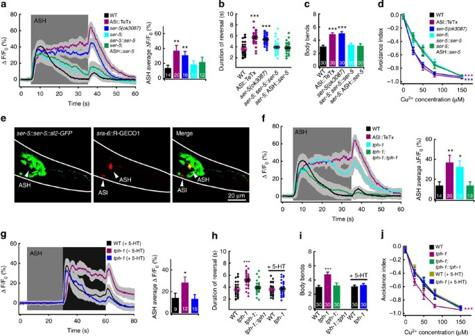Figure 3: 5-HT and the SER-5 receptor transduce ASI inhibition of ASHs. (a) ASH calcium responses to 10 mM CuSO4in wild-type, ASI neurotransmission blocked,ser-5mutant, andser-5p::ser-5and ASH::ser-5genetically rescued worms. Summation of the kinematics of Cu2+avoidance behaviours (b,c) and Cu2+sensitivity (d,n≥8 assays) in the worms mentioned above. (e) The expression pattern ofser-5p::ser-5::sl2-GFPandsra-6p::R-GECO1inser-5-null mutants. These genes were co-expressed in ASH neurons. Scale bar, 20 μm. (f) Thetph-1lof mutation had a similar effect on the ASH Cu2+-elicited Ca2+signals as did genetically silencing ASI with TeTx, and the defect was rescued bytph-1p::tph-1ectoexpression. (g) The defect of the ASH Ca2+transients in thetph-1mutants was rescued by application of 5 mM exogenous 5-HT. Summation of the kinematics of Cu2+avoidance behaviours (h,i) and Cu2+sensitivity (j,n≥8 assays) in the worms denoted. All data are expressed as means±s.e.m. The number on each bar indicates the number of independent tests for each genotype. One-way analysis of variance (ANOVA) test ina–candf–i, and two-way ANOVA test indandj. Corrected with Bonferronit-test. Values that differ significantly are indicated (*P≤0.05, **P≤0.01 and ***P≤0.001 compared with the wild-type N2 control). Figure 3: 5-HT and the SER-5 receptor transduce ASI inhibition of ASHs. ( a ) ASH calcium responses to 10 mM CuSO 4 in wild-type, ASI neurotransmission blocked, ser-5 mutant, and ser-5p::ser-5 and ASH ::ser-5 genetically rescued worms. Summation of the kinematics of Cu 2+ avoidance behaviours ( b , c ) and Cu 2+ sensitivity ( d , n ≥8 assays) in the worms mentioned above. ( e ) The expression pattern of ser-5p::ser-5::sl2-GFP and sra-6p::R-GECO1 in ser-5 -null mutants. These genes were co-expressed in ASH neurons. Scale bar, 20 μm. ( f ) The tph-1 lof mutation had a similar effect on the ASH Cu 2+ -elicited Ca 2+ signals as did genetically silencing ASI with TeTx, and the defect was rescued by tph-1p::tph-1 ectoexpression. ( g ) The defect of the ASH Ca 2+ transients in the tph-1 mutants was rescued by application of 5 mM exogenous 5-HT. Summation of the kinematics of Cu 2+ avoidance behaviours ( h , i ) and Cu 2+ sensitivity ( j , n ≥8 assays) in the worms denoted. All data are expressed as means±s.e.m. The number on each bar indicates the number of independent tests for each genotype. One-way analysis of variance (ANOVA) test in a – c and f – i , and two-way ANOVA test in d and j . Corrected with Bonferroni t -test. Values that differ significantly are indicated (* P ≤0.05, ** P ≤0.01 and *** P ≤0.001 compared with the wild-type N2 control). Full size image ADFs act as interneurons to mediate ASI inhibiting ASHs Among serotoninergic neurons, NSMs, AIMs and RIH showed no Cu 2+ -evoked Ca 2+ signals in wild-type and ASI-blocked worms ( Supplementary Fig. 4a–c ). Only ADF neurons showed a Cu 2+ -evoked Ca 2+ response. Furthermore, the onset of the Ca 2+ signals was delayed by silencing ASIs ( Fig. 4a ), suggesting that ADFs probably relayed ASI inhibition to ASHs. To validate the ADF intermediate function, we examined the impact of optogenetically inhibiting ASIs on Cu 2+ -evoked Ca 2+ signals of ADFs. As expected, the Ca 2+ response in ADFs was significantly delayed by specific optogenetic inhibition of ASIs, but the intensity was not altered ( Fig. 4a ). We further employed unc-13 lof mutation to validate the observation. As the gene unc-13 is essential for synaptic vesicle exocytosis and neurotransmitter release [39] , [40] , the lof mutants were used to analyse the sensational response in sensory neurons under neuronal isolation [41] , [42] . Our data showed the lof mutation of unc-13 ( e1091 ) had a similar impact on ADF Cu 2+ -elicited Ca 2+ transients to genetically blocking or optogenetically inhibiting ASIs ( Fig. 4b ), suggesting that sensory ADF neurons may probably be sensitive to Cu 2+ . We then tested whether artificial activation of ASI promotes a more rapid onset of the Ca 2+ response in ADFs. Unexpectedly, chemogenetic activation of ASIs with 100 μM capsaicin had no apparent impact on the Ca 2+ signals in ADFs with ( Supplementary Fig. 4d , 5–30 s) or without ( Supplementary Fig. 4d , 30–60 s) the Cu 2+ stimulation. Prolonged direct chemogenetic activation of ADFs (55 s) without CuSO 4 resulted in no apparent ADF Ca 2+ transients in the ASI-blocked worms and very slowly appearing Ca 2+ transients in the ASI-undisrupted worms ( Supplementary Fig. 4e ). In addition, chemogenetically activating ADFs evoked no apparent Ca 2+ signal without the Cu 2+ stimulation ( Supplementary Fig. 4f , 5–30 s), and did not change the ASI promotion of ADF Cu 2+ -evoked Ca 2+ signals, if compared the delay time and amplitude of their Ca 2+ signals ( Supplementary Fig. 4f , 30–60 s) with those in the ADF-undisturbed worms ( Fig. 4a ). These results suggest that ASIs do not directly activate ADFs, but instead permit a more rapid onset of Cu 2+ -elicited Ca 2+ responses in ADFs and also support that ADFs are Cu 2+ sensitive. 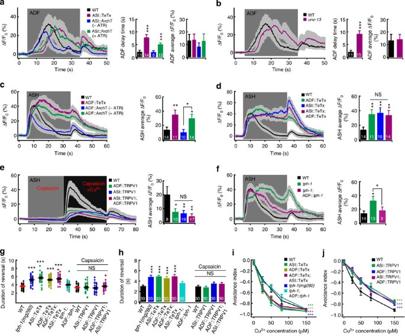Figure 4: ADF neurons mediate ASI inhibition of ASHs. ADF Ca2+responses to the 10 mM CuSO4stimulation in the ASI-silenced and ASI-opto-inhibited worms (a), andunc-13mutants (b). The delay time was calculated as the time of stimulus application to the time when the single-exponential fitted curve of individual Ca2+on-response trace cuts fitted straight line of basal Ca2+signals before stimulation. (c) Genetically blocking and optogenetically inhibiting ADF neurons similarly prolonged the ASH Cu2+-evoked Ca2+signals. Silencing ASIs, ADFs and both types of neurons with TeTx had similar effects on the ASH Cu2+-elicited Ca2+transients (d) and chemogenetically activating ASIs, ADFs and both types of neurons also had the similar effects on the ASH Ca2+signals (e). The neuron expressing rat TRPV1 cation channels was activated by the application of 100 μM capsaicin. (f) ASH Ca2+response to the 10 mM Cu2+stimulation intph-1mutants and in ADF::tph-1genetically rescued worms. The durations (g) and body bends (h) of the Cu2+-evoked reversal in wild-type N2 and the neuronal manipulated worms assayed by the dry drop test. (i) Similar effects on animal Cu2+sensitivity were observed amongtph-1lof mutation that were rescued by its ADF expression, genetically silencing and optogenetically inhibiting ASIs, ADFs and both types of neurons (n≥8 assays). (j) Chemogenetically activating ASIs, ADFs and both types of neurons had similar effects on animal Cu2+sensitivity (n≥8 assays). All data are expressed as means±s.e.m. The number on each bar indicates the number of independent tests for each genotype. One-way analysis of variance (ANOVA) test ina–hand two-way ANOVA test iniandj. Corrected with Bonferronit-test. Values that differ significantly are indicated (*P≤0.05, **P≤0.01 and ***P≤0.001; n.s., not significant compared with the wild-type N2 control or as indicated). Figure 4: ADF neurons mediate ASI inhibition of ASHs. ADF Ca 2+ responses to the 10 mM CuSO 4 stimulation in the ASI-silenced and ASI-opto-inhibited worms ( a ), and unc-13 mutants ( b ). The delay time was calculated as the time of stimulus application to the time when the single-exponential fitted curve of individual Ca 2+ on-response trace cuts fitted straight line of basal Ca 2+ signals before stimulation. ( c ) Genetically blocking and optogenetically inhibiting ADF neurons similarly prolonged the ASH Cu 2+ -evoked Ca 2+ signals. Silencing ASIs, ADFs and both types of neurons with TeTx had similar effects on the ASH Cu 2+ -elicited Ca 2+ transients ( d ) and chemogenetically activating ASIs, ADFs and both types of neurons also had the similar effects on the ASH Ca 2+ signals ( e ). The neuron expressing rat TRPV1 cation channels was activated by the application of 100 μM capsaicin. ( f ) ASH Ca 2+ response to the 10 mM Cu 2+ stimulation in tph-1 mutants and in ADF:: tph-1 genetically rescued worms. The durations ( g ) and body bends ( h ) of the Cu 2+ -evoked reversal in wild-type N2 and the neuronal manipulated worms assayed by the dry drop test. ( i ) Similar effects on animal Cu 2+ sensitivity were observed among tph-1 lof mutation that were rescued by its ADF expression, genetically silencing and optogenetically inhibiting ASIs, ADFs and both types of neurons ( n ≥8 assays). ( j ) Chemogenetically activating ASIs, ADFs and both types of neurons had similar effects on animal Cu 2+ sensitivity ( n ≥8 assays). All data are expressed as means±s.e.m. The number on each bar indicates the number of independent tests for each genotype. One-way analysis of variance (ANOVA) test in a – h and two-way ANOVA test in i and j . Corrected with Bonferroni t -test. Values that differ significantly are indicated (* P ≤0.05, ** P ≤0.01 and *** P ≤0.001; n.s., not significant compared with the wild-type N2 control or as indicated). Full size image We expected that manipulating ADFs would have the same effects on the ASH calcium transients and worm Cu 2+ -elicited avoidance behaviours as did manipulating ASIs. Indeed, as anticipated, blocking or inhibiting ADF neurotransmission by TeTx or ArchT, significantly enhanced ASH Ca 2+ signals ( Fig. 4c ), and blocking ADFs, ASIs and both pairs of neurons had no significant difference in their effects on the ASH Ca 2+ signals ( Fig. 4d ). Chemogenetically activating ASIs, ADFs and both types of neurons with only the application of capsaicin had no effect on Cu 2+ -unstimulated ASHs ( Fig. 4e , 5–30 s), but inhibited ASH Cu 2+ -evoked Ca 2+ responses similarly ( Fig. 4e , 30–60 s). These results confirm that ADFs mediate the ASI inhibition of ASHs. The tph-1 lof mutation was expected to have a similar effect on ASH Cu 2+ -elicited Ca 2+ signals as did blocking ASI and should be rescued by the expression of the gene in ASHs. As expected, tph-1 ( mg280 ) mutants showed an augmented Ca 2+ transient and the defect was rescued by the specific expression of tph-1 in ADF neurons ( Fig. 4f ). Furthermore, inhibition of ADFs, ASIs, both types of neurons and the tph-1 lof mutation had very similar effects on aversive behaviours tested by the dry drop and the worm Cu 2+ sensitivities assayed by the quadrant assay ( Fig. 4g–i and Supplementary Fig. 4g ). In addition, chemogenetically activating ADFs, ASIs and both types of neurons also had similar effects on Cu 2+ avoidance and Cu 2+ sensitivity ( Fig. 4g,h,j and Supplementary Fig. 4h ). ADFs are postsynaptic neurons of ASHs ( www.wormweb.org ) and they may receive neural signals directly from ASHs. We then positively ( Supplementary Fig. 5a ) and negatively manipulated ASH neurons and examined the changes of Ca 2+ transients in ADFs to test the hypothesis. Chemogenetic activation of ASHs with TRPV1 plus capsaicin did not change ADF activity ( Supplementary Fig. 5b ). Permanently blocking ASHs with TeTx, optogenetically inhibiting ASH with ArchT and chemogenetically inhibiting ASHs with the Drosophila HisCl1 channel [43] plus 30 mM histamine also had no effect on Cu 2+ -elicited Ca 2+ transients in ADFs ( Supplementary Fig. 5c–h ). Moreover, blocking both ASIs and ASHs had a similar effect on ADF Cu 2+ -evoked Ca 2+ signals to blocking ASI alone ( Supplementary Fig. 5i,j ). These results exclude the possibility that ADFs receive neural signals from ASHs, which then feed back to inhibit ASHs. Taken together, ASIs advance sensory serotonergic ADF excitation to release the neurotransmitter 5-HT that inhibits ASH neurons during the Cu 2+ stimulation. ASIs are neuropeptidergic neurons ( www.wormatlas.org ). To test whether neuropeptides mediate the neurotransmission between ASIs and ADFs, we used mutants that have defects in neuropeptide release and biogenesis. unc-31 is necessary for neuropeptide release from dense cored vesicles [44] , [45] . In unc-31 ( e928 ) mutants, ADFs showed a delayed onset of Cu 2+ -evoked Ca 2+ transients ( Supplementary Fig. 6a ). The egl-3 gene encodes a homologue of a mammalian proprotein convertase that participates in peptide secretion [46] and the egl-21 gene encodes a putative carboxypeptidase that is required for normal synthesis of FMRFamide-like peptides and neuropeptide-like peptides [47] . Our data showed that the lof mutations of egl-3 ( egl-3 ( tm1377 )) and egl-21 ( egl-21 ( n476 )) postponed the ADF Ca 2+ signals ( Supplementary Fig. 6b ). We also observed significant defects in the ADF Ca 2+ signals in nlp-5 , ins-1 and ins-3 mutants ( Supplementary Fig. 6c ). These data suggest that neuropeptides most probably mediate the neurotransmission between ASIs and ADFs. Altogether, our results strongly support that sensory ASI neurons sense Cu 2+ and permit ADFs to accelerate the onset of ADF activity during the Cu 2+ stimulation for 30 s. Sensory ADF neurons sense Cu 2+ stimulation and release 5-HT to inhibit ASHs. SER-3 receptor intermediates ASH inhibiting ASIs Direct activations of ASIs by photogenetic stimulation with ChR2 (ref. 6 ) and a high K + solution [42] evoke continuously increasing Ca 2+ signals other than only an off- but no obvious on-response of Cu 2+ -evoked Ca 2+ transients under physiological condition, suggesting that ASI neurons receive inhibitory signals from other neurons. ASIs inhibit ASHs during Cu 2+ stimulation, but whether ASHs inhibit ASIs to form a reciprocal inhibition circuit remained unclear. To answer this question, we first examined the effects of blocking ( Fig. 5a ) and inhibiting ASHs on Cu 2+ -elicited Ca 2+ signals in ASIs. Our results showed that permanently blocking or temporarily opto-inhibiting ASHs resulted in an obvious on-response of Cu 2+ -evoked Ca 2+ signals in ASIs ( Fig. 5b and Supplementary Movie 9 ). As expected, ASH Cu 2+ -elicited Ca 2+ signals were reduced by opto-inhibition with ArchT but were not disturbed by the permanent block with TeTx ( Supplementary Fig. 7a ). These results suggest that the ASI on-response is inhibited by ASHs. 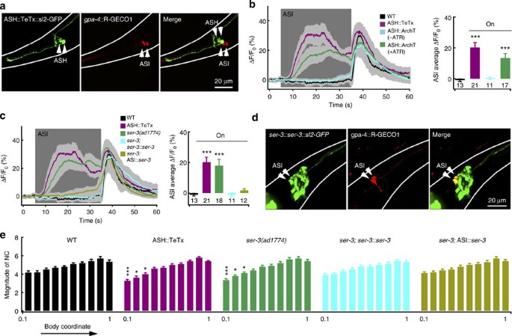Figure 5: Octopamine and the SER-3 receptor transduce ASH inhibition to ASIs. (a) The specific expression of TeTx in ASH neurons achieved by the use of FLP–FRT site-specific recombination system and R-GECO1 in ASI neurons directed by thegpa-4promoter. Scale bars, 20 μm. (b) Genetically silencing and optogenetically inhibiting ASHs resulted in a big on-response of Cu2+-evoked Ca2+response in ASI neurons. (c) Theser-3lof mutation had a similar effect on the ASI response to the 10 mM CuSO4stimulation as silencing ASHs with TeTx, which could be rescued by extrachromosomal expression of the gene driven by its own or an ASI-specific promoter. (d) The expression patterns ofser-3p::ser-3::sl2-GFPandgpa-4p::R-GECO1inser-3-null animals. These genes were co-expressed in ASI neurons. (e) The bending magnitude of the Cu2+avoidance in wild type, mutant and transgenic worms (n=30 assays). All data are expressed as means±s.e.m. The number on each bar indicates the number of independent tests for each genotype. One-way analysis of variance (ANOVA) test inb,cand two-way ANOVA test ine. Corrected with Bonferronit-test. Values that differ significantly are indicated (*P≤0.05, **P≤0.01 and ***P≤0.001 compared with the wild-type N2 control). Figure 5: Octopamine and the SER-3 receptor transduce ASH inhibition to ASIs. ( a ) The specific expression of TeTx in ASH neurons achieved by the use of FLP–FRT site-specific recombination system and R-GECO1 in ASI neurons directed by the gpa-4 promoter. Scale bars, 20 μm. ( b ) Genetically silencing and optogenetically inhibiting ASHs resulted in a big on-response of Cu 2+ -evoked Ca 2+ response in ASI neurons. ( c ) The ser-3 lof mutation had a similar effect on the ASI response to the 10 mM CuSO 4 stimulation as silencing ASHs with TeTx, which could be rescued by extrachromosomal expression of the gene driven by its own or an ASI-specific promoter. ( d ) The expression patterns of ser-3p::ser-3::sl2-GFP and gpa-4p::R-GECO1 in ser-3 -null animals. These genes were co-expressed in ASI neurons. ( e ) The bending magnitude of the Cu 2+ avoidance in wild type, mutant and transgenic worms ( n =30 assays). All data are expressed as means±s.e.m. The number on each bar indicates the number of independent tests for each genotype. One-way analysis of variance (ANOVA) test in b , c and two-way ANOVA test in e . Corrected with Bonferroni t -test. Values that differ significantly are indicated (* P ≤0.05, ** P ≤0.01 and *** P ≤0.001 compared with the wild-type N2 control). Full size image ASHs are postsynaptic but not presynaptic cells of ASIs [48] . Therefore, it is likely to be that ASH neurons modulate ASIs via a mediator. We then explored the molecular mechanism underlying the ASH inhibiting ASIs, employing the same strategy used in identifying the SER-5 receptor. We found that ASI Ca 2+ on-responses in ser-1 ( ok345 ), ser-3 ( ad1774 ), ser-3 ( ok1995 ) and tyra-2 ( tm1815 ) mutants were similar to those in the ASH-silenced worms ( Supplementary Fig. 8 ), but only ser-3 mutants were rescued by extrachromosomal expression of the gene driven by its own or an ASI-specific promoter ( Fig. 5c ). These results suggest ser-3 probably mediated the ASH inhibition of ASIs. The gene ser-3 encodes an OA receptor that is widely expressed in a number of head and tail neurons including ASIs [14] ( Fig. 5d ). The Cu 2+ evoked avoidance behaviour and Cu 2+ sensitivity in ser-3 mutants were also similar to those in the ASH-blocked worms, and were rescued by its own or an ASI-specific promoter ( Fig. 5e and Supplementary Fig. 7b–d ). These data suggest that SER-3 directly functions in ASI neurons to mediate the ASH inhibition of ASIs. Octopaminergic RIC neurons mediate ASH inhibiting ASIs Because ser-3 encodes an OA receptor, we next tested whether OA is the ligand that mediates the ASH inhibition of ASIs. We checked the tbh-1 ( n3247 ) mutants that are unable to biosynthesize OA [49] , [50] . In the mutants, the Cu 2+ -elicited on-response of Ca 2+ signals in ASIs was significantly augmented, although the amplitudes were smaller than those observed in the ASH-blocked worms ( Fig. 6a,b ). Specific expression of tbh-1 driven by its own promoter in RIC neurons fully rescued the defects in the ASI Ca 2+ signals ( Fig. 6a ). As RICs have no synaptic connection with ASIs [48] , RICs probably function as neuroendocrine cells to mediate the ASH inhibition of ASIs. 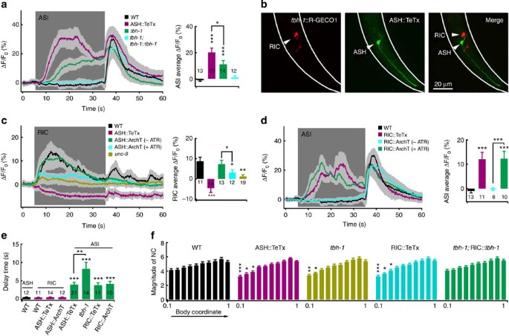Figure 6: RIC neurons mediate the inhibition of ASIs by ASHs. (a) ASI Ca2+responses to the 10 mM Cu2+stimulation in wild-type, ASH silenced,tbh-1mutant andtbh-1p::tbh-1rescued worms. (b) The expression of R-GECO1 in RIC neurons driven bytbh-1promoter and the specific expression of TeTx in ASH neurons realized by the use of the FLP–FRT site-specific recombination system. Scale bar, 20 μm. (c) Permanently or temporarily silencing ASH neurons with TeTx or ArchT had a similar effect on RIC Ca2+responses to the 10 mM CuSO4stimulation. (d) ASIs showed an obvious on-response of Cu2+-elicited Ca2+signals after blocking or inhibiting RICs. (e) The delay time of Cu2+-evoked calcium transients of ASH, RIC and ASI neurons in worms indicated. The delay time was calculated as the time of stimulus application to the time when the single-exponential fitted curve of individual Ca2+on-response trace cuts fitted straight line of basal Ca2+signals before stimulation. (f) The bending magnitude of Cu2+-evoked reversals in wild type, mutant and transgenic worms (n=30 assays). All data are expressed as means±s.e.m. The number on each bar indicates the number of independent tests for each genotype. One-way analysis of variance (ANOVA) test inaandc–e, and two-way ANOVA test inf. Corrected with Bonferronit-test for multiple comparisons. Values that differ significantly are indicated (*P≤0.05, **P≤0.01 and ***P≤0.001 compared with the wild-type N2 control). Figure 6: RIC neurons mediate the inhibition of ASIs by ASHs. ( a ) ASI Ca 2+ responses to the 10 mM Cu 2+ stimulation in wild-type, ASH silenced, tbh-1 mutant and tbh-1p::tbh-1 rescued worms. ( b ) The expression of R-GECO1 in RIC neurons driven by tbh-1 promoter and the specific expression of TeTx in ASH neurons realized by the use of the FLP–FRT site-specific recombination system. Scale bar, 20 μm. ( c ) Permanently or temporarily silencing ASH neurons with TeTx or ArchT had a similar effect on RIC Ca 2+ responses to the 10 mM CuSO 4 stimulation. ( d ) ASIs showed an obvious on-response of Cu 2+ -elicited Ca 2+ signals after blocking or inhibiting RICs. ( e ) The delay time of Cu 2+ -evoked calcium transients of ASH, RIC and ASI neurons in worms indicated. The delay time was calculated as the time of stimulus application to the time when the single-exponential fitted curve of individual Ca 2+ on-response trace cuts fitted straight line of basal Ca 2+ signals before stimulation. ( f ) The bending magnitude of Cu 2+ -evoked reversals in wild type, mutant and transgenic worms ( n =30 assays). All data are expressed as means±s.e.m. The number on each bar indicates the number of independent tests for each genotype. One-way analysis of variance (ANOVA) test in a and c – e , and two-way ANOVA test in f . Corrected with Bonferroni t -test for multiple comparisons. Values that differ significantly are indicated (* P ≤0.05, ** P ≤0.01 and *** P ≤0.001 compared with the wild-type N2 control). Full size image TA is an intermediate in the synthesis of OA [49] , [50] . To test whether TA has the same function as OA, we used tdc-1 ( n3419 ) mutants that fail to biosynthesize both TA and OA. We examined the Cu 2+ -evoked avoidance behaviour in the mutants. Our data showed that the tdc-1 ( n3419 ) worms exhibited the similar defects in the Cu 2+ -evoked aversive behaviour and Cu 2+ sensitivity to the tbh-1 mutants ( Supplementary Fig. 9a–d ), suggesting that TA did not probably mediate the ASH modulation of ASIs. ASH neurons connect with RICs by gap junctions [48] . To further confirm the intermediate function of RICs in ASH inhibiting ASIs, we employed TeTx ( Fig. 6b ) to permanently block ASH neurotransmission, or ArchT to optogenetically inhibit ASHs. Our results showed that the Ca 2+ transients of RICs were significantly reduced in ASH-inhibited worms and even reversed in the ASH-blocked animals ( Fig. 6c ). The gene unc-9 encodes an innexin, an integral transmembrane channel protein that is a structural component of invertebrate gap junctions, which is expressed in RICs [51] ( Supplementary Fig. 9e ). The unc-9 mutation ( unc-9 ( e101 )) had similar effect on RIC Cu 2+ -elicited Ca 2+ signals as did the negative manipulation of ASHs with TeTx and ArchT ( Fig. 6c ). In addition, the lof mutation of another innexin encoding gene inx-4 (in inx-4(e1128 )) had a similar phenotype to the unc-9 mutation ( Supplementary Fig. 9f ). These data suggest that permanent expression of TeTx most probably disrupts neurotransmission through the gap junctions. Direct manipulation of RICs would have the same effect on ASI Cu 2+ -evoked Ca 2+ signals as manipulating ASHs. Indeed, negative manipulation of RICs with TeTx and ArchT affected the ASI Ca 2+ transients ( Fig. 6d and Supplementary Fig. 9g ) similar to blocking and inhibiting ASHs ( Fig. 5b ). In addition, the RIC calcium responses to Cu 2+ were synchronized with those of ASHs ( Fig. 6e ). More importantly, our analysis of worm Cu 2+ avoidance behaviour and Cu 2+ sensitivity ( Fig. 6f and Supplementary Fig. 9h–j ) confirmed the conclusion derived from the Ca 2+ data. Altogether, these data support that RICs connect postsynaptically with ASHs and are excited directly by ASHs, and that RICs release OA that directly acts on SER-3 in ASIs to mediate the ASH inhibition of ASIs. Cross-inhibitory neural circuitry between ASHs and ASIs We hereby determine that ASI and ASH sensory neurons inhibit reciprocally, and the neurotransmitters 5-HT (released by ADFs) and OA (released by RICs) transduce neuronal signals from these two pairs of sensory neurons by binding their receptors SER-5 and SER-3, respectively. We then used a ser-5 ; ser-3 double mutation ( ser-3(ad1774) I; ser-5(ok3087) I ) and genetically blocked both ASHs and ASIs, to further confirm the roles of SER-5 and SER-3 signalling pathways in the modulation of Cu 2+ -elicited Ca 2+ responses in ASHs and ASIs, as well as worm Cu 2+ -evoked aversive behaviour. As expected, the double mutation of ser-3 and ser-5 affected Cu 2+ -elicited Ca 2+ signals of ASH and ASI neurons ( Fig. 7a,b and Supplementary Movie 10 ) similar to the silencing of both ASIs and ASHs ( Fig. 7a,b and Supplementary Movie 11 ). Fortunately, we were able to occasionally record calcium signals in both ASIs and ASHs at the same focal plane of the objective lens ( Supplementary Movies 10 and 11 ), which directly visualized the Ca 2+ signals of both ASIs and ASHs in the double-blocked worms. We further analysed the avoidance behaviour in the double mutants. Our data showed that the double mutants exhibited similar behavioural defects tested by the dry drop assay to those in the double-silenced worms ( Fig. 7c–e and Supplementary Movies 5 and 12 ). These results suggest that the cross-inhibition between ASHs and ASIs is transduced primarily by 5-HT and OA signalling pathways. We did not examine the Cu 2+ sensitivity in the double mutants and the double-silenced worms tested by the quadrant assay, as these worms were seriously uncoordinated. Altogether, our study demonstrates that a cross-inhibitory circuit exists between ASH and ASI sensory neurons, which modulates the Cu 2+ nociception and drives an adaptive avoidance behaviour. The synaptic connections, functional actions and underlying signalling pathways among neurons in the circuit, and the function of the reciprocal inhibition in nociception and aversive behaviour, are summarized in Fig. 7f,g . 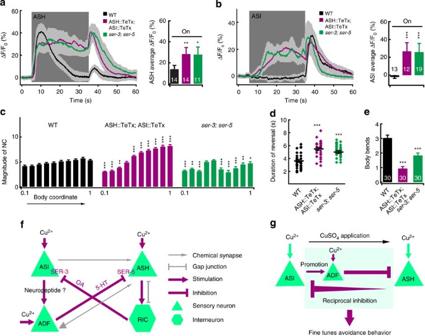Figure 7: A dynamic reciprocal inhibition between ASHs and ASIs, and the neuronal circuit. Theser-3; ser-5double mutation had a similar effect on ASH (a) and ASI (b) calcium responses to the 10 mM CuSO4stimulation as did silencing both the ASH and ASI neurons. (c) The bending magnitude along the body centre line in both the ASH and ASI neurons silenced worms andser-3; ser-5double mutants (n=30 assays). The durations (d) and body bends (e) of the Cu2+-evoked reversals assayed by the dry drop test in worms are indicated. (f) Synaptic connections, functional actions and the underlying signalling pathways among neurons in the ASI–ASH reciprocal inhibitory neuron circuit. (g) Schematic representation of the cross-inhibition between sensory neuron ASHs and ASIs that fine-tunes nociception and avoidance behaviour. All data are expressed as means±s.e.m. The number on each bar indicates the number of independent tests for each genotype. One-way analysis of variance (ANOVA) test ina,bandd,e, and two-way ANOVA test inc. Corrected with Bonferronit-test for multiple comparisons. Values that differ significantly are indicated (*P≤0.05, **P≤0.01 and ***P≤0.001 compared with the wild-type N2 control). Figure 7: A dynamic reciprocal inhibition between ASHs and ASIs, and the neuronal circuit. The ser-3; ser-5 double mutation had a similar effect on ASH ( a ) and ASI ( b ) calcium responses to the 10 mM CuSO 4 stimulation as did silencing both the ASH and ASI neurons. ( c ) The bending magnitude along the body centre line in both the ASH and ASI neurons silenced worms and ser-3; ser-5 double mutants ( n =30 assays). The durations ( d ) and body bends ( e ) of the Cu 2+ -evoked reversals assayed by the dry drop test in worms are indicated. ( f ) Synaptic connections, functional actions and the underlying signalling pathways among neurons in the ASI–ASH reciprocal inhibitory neuron circuit. ( g ) Schematic representation of the cross-inhibition between sensory neuron ASHs and ASIs that fine-tunes nociception and avoidance behaviour. All data are expressed as means±s.e.m. The number on each bar indicates the number of independent tests for each genotype. One-way analysis of variance (ANOVA) test in a , b and d , e , and two-way ANOVA test in c . Corrected with Bonferroni t -test for multiple comparisons. Values that differ significantly are indicated (* P ≤0.05, ** P ≤0.01 and *** P ≤0.001 compared with the wild-type N2 control). Full size image In the present study, we find that sensory neuron ASIs modulate the ASH Cu 2+ reception and worm Cu 2+ -aversive behaviours by cross-inhibition with ASHs, and we dissect the neural circuit and molecular mechanism as shown in Fig. 7f . In this neuronal circuit, ASHs respond to the nociceptive Cu 2+ stimulus quickly and robustly, which allows ASHs to predominate over and inhibit ASIs at the initial stage. ASI sensory neurons are secondary Cu 2+ sensory neurons, because they have a weaker Cu 2+ response. ASI probably release neuropeptides in a state of undetectable Cu 2+ -induced Ca 2+ signals in the soma to permit and promote a more rapid onset of Cu 2+ -evoked activity in ADFs. ADFs are also sensitive to Cu 2+ , but their activities need permission and promotion from ASIs. Permitted by ASIs and stimulated by Cu 2+ , ADFs release 5-HT to inhibit ASHs by binding SER-5. The positive and negative manipulation of ASIs, ADFs and both the two pairs of neurons have similar effects on Cu 2+ -evoked Ca 2+ signals of ASHs and worm Cu 2+ -aversive behaviour; besides, the phenotypes of the tph-1 mutants that have a defect in 5-HT biosynthesis is rescued by ADF-specific expression of the gene ( Fig. 4 ). These data strongly support that ASI→ADF→5-HT→ASH is a major pathway mediating ASI inhibition of ASHs. However, these data can not completely rule out that ASI could affect ASH by additional pathways. ASI functions as a modulator to suppress hyper-nociception and fine-tune worm avoidance behaviour. This circuit is similar to the central flip-flop circuit that integrates contradictory sensory cues in C. elegans feeding regulation [52] . However, there are differences between the two circuits: (1) the central feeding regulatory circuit integrates two different sets of sensory information from the olfactory attractive cues and the gustatory or the olfactory repellents, whereas the peripheral circuit receives the same sensory information from gustatory nociceptive stimuli; (2) the kinetics of the two circuits are different, as the peripheral circuit is biased and progress dependent, whereas the central circuit is bistable and fast switchable, although the nociceptive sensory information has more effects than that of attraction; and (3) their functions are different, in that the central circuit functions to make a rapid decision, whereas the peripheral circuit fine-tunes nociceptive sensation and suppress hyper-responding behaviour. ASIs inhibit ASHs through the intermediation of ADF sensory neurons that function as interneurons, similar to the functional metamorphosis of AWC ON sensory neuron in the salt sensation circuit [41] . To date, there is no report that shows ADFs are Cu 2+ sensitive. ADFs are post-synaptic to 8 cells: AWBs (11, the number of synapses) that mediate avoidance to 2-nonanone and 1-octanol, ASHs (5), AWAs (3) that mediate chemotaxis to diacetyl, pyrazine and trimethylthiazole [53] , ASEs (1) that mediate avoidance behaviour from Cd 2+ and Cu 2+ ion [54] , and interneurons AVHs (3), AIYs (1), PVPs (1) and RIH (1). ADF Ca 2+ signals during CuSO 4 stimulation may be a result of neurotransmission from their synaptically connected neuron, particularly from ASHs and ASEs, in addition to the ASIs we identified. However, permanently silencing, opto- and chemo-inhibiting and chemo-activating ASHs had no effect on the ADF Ca 2+ signals ( Supplementary Fig. 5a–h ); silencing both ASHs and ASIs postpones the onset of the ADF Ca 2+ signals similar to blocking ASIs alone ( Supplementary Fig. 5i,j ); the unc-13 lof mutation delays the ADF Ca 2+ onset similar to silencing or inhibiting ASIs ( Fig. 4a,b ); and with silenced ASIs, CuSO 4 evokes Ca 2+ transients much more efficiently than the chemogenetical activation in ADFs ( Supplementary Fig. 4e,f ). Collectively, these data show that ADFs receive excitation from ASIs but not from ASHs and are sensitive to Cu 2+ stimulation, although the detection mechanism needs to be identified. In addition, our data show that ASIs play permission role to promote a more rapid onset of the response in ADF most probably through the intermediation of neurohormonal peptides ( Supplementary Fig. 6 ). Interestingly, why the worm does not employ an ASH→ADF→5-HT→ASH feedback is unclear. We suspect that, first, in a small organism such as C. elegans or in a small local area, neuroendocrine is effective as chemical synaptic neurotransmission, especially for the slow kinetic process of sensory modulation. Second, sensational modulation by cross-inhibition using two or multi-information inputs is more adaptive than negative feedback using only one information input. In this work, our data show the ASI neurotransmission in undetectable increases in the soma cytosolic Ca 2+ levels plays a key role in the reciprocal inhibition. Many sensory neurons do not fire action potentials in response to stimuli. Graded release of neurotransmitters is widely used in sensory neurons, including photoreceptor cells [55] , auditory hair cells [56] and olfactory neurons [57] . In C. elegans , AWC neurons have non-spiking, have tonic neurotransmitter release at rest and respond to excitatory or inhibitory inputs with graded changes in membrane potential and transmitter release [57] . The possibly tonic neurotransmitter release at rest and graded transmitter release during the stimulation in ASIs need further investigation. In this study, we use embryonic expression of the clostridial neurotoxin TeTx to permanently block neurotransmission. TeTx is a specific protease of synaptobrevin. The vesicular SNARE protein synaptobrevin is essential for neurotransmitter release and exocytosis of dense-core vesicles [58] , [59] . Our data show that silencing ASHs with embryonic expression of TeTx has even more significant effects on RIC Ca 2+ signals than opto-inhibiting ASHs and lof mutation of innexin encoding genes unc-9 ( Fig. 6c ) and inx-4 ( Supplementary Fig. 9f ). As there are only gap junctions between ASHs and RICs, these results show embryonic and permanent expression of TeTx not only disrupts the neurotransmitter release via synaptic vesicle fusion with the plasma membrane, but also blocks transmission through gap junctions. One possible explanation is that innexin traffic to the plasma membrane via dense-core vesicles, which is essential for the formation of gap junctions, is interrupted by the permanent expression of the neurotoxin TeTx. Inducible expression of TeTx in adults is needed to resolve this issue. The gene tdc-1 encodes the major C. elegans tyrosine decarboxylase that is necessary for TA biosynthesis, and tbh-1 encodes a putative dopamine β-hydroxylase that transforms TA into OA [49] , [50] . OA and TA have been reported to function independently to modulate many behaviours [14] , [15] , [49] , [50] . In this study, we did not observe more serious defects in the tdc-1 mutants compared with tbh-1- mutated worms. However, our current data are not conclusive enough to exclude the possibility that TA functions in the regulation of the Cu 2+ -elicited aversive behaviours. Another possible explanation is that TA and OA act antagonistically in response to a Cu 2+ stimulus as previously suggested [60] . A third hypothesis is that OA biosynthesis in the tdc-1(n3419) II mutant may be not fully blocked. Sensory neurons can be modulated by central and peripheral nervous systems. Peripheral modulations of sensation exist universally in various sensory modalities, including pain, vision and hearing. Disorders of sensory modulation cause diseases. The ASI modulation of ASH-mediated nociception in C. elegans determined by this work suppresses the super sensation and super behavioural responses. Our work paves the way to better understand peripheral modulations of the sensations in other animals, including humans. Strains The C. elegans strains used in this study are listed in Supplementary Table 1 . All strains were maintained and grown according to the standard procedures [49] . The double mutant animals were generated using the standard genetic techniques and confirmed by PCR and sequencing. Most constructs were injected at 30 ng μl −1 together with lin44p::GFP (5 ng μl −1 ) as a co-injection marker using the standard techniques. At least five independent lines were examined for each rescue experiment and in vivo calcium imaging. Construction of plasmids and entry clones Three-Fragment Multisite gateway (Invitrogen, Thermo Fisher Scientific, Waltham, MA, USA) and In-Fusion (Clontech Laboratories, Inc., Mountain View, CA, USA) technology were used to generate the constructs used in this study. Briefly, three entry clones comprising three PCR products (promoter, gene of interest, sl2-GFP or 3′UTR , in name of slot1, slot2 and slot3, respectively) were recombined into the pDEST R4-R3 Vector II or custom-modified destination vectors using att L- att R (LR) recombination reactions to generate the expression clones. To construct the slot1 entry clone, the att B4-stop- att B1r PCR product was recombined with the att P4 and att P1r sites in the pDONR-P4-P1R vector using the att B- att P (BP) recombination reactions. A modified vector containing att L4-stop- att R1 fragment used for the LR recombination reactions was generated. The promoters such as sra-6p , gpa-4p , gpa-11p , ser-5p , tph-1p , srh-142p , ceh-2p , mod-5p , ser-3p and tbh-1p were PCR amplified from wild-type N2 genomic DNA and used to substitute for the –stop– fragment in the modified donor vector with the in-fusion method to generate the slot1 entry clones. The length of sra-6p , gpa-4p , gpa-11p , srh-142p , ceh-2p , mod-5p , ser-5p , tph-1p , ser-3p , tbh-1p and unc-9p are 3.8, 2.5, 3.3, 3.5, 1.6, 4.2, 3.5, 3.7, 2, 4.6 and 2 kb, respectively. To generate the entry clones slot2 and slot3, we used BP recombination reactions. The ser-5 , ser-3 and tph-1 were PCR amplified from C. elegans N2 worm genomic DNA and tbh-1a complementary DNA was amplified by PCR with primers containing att B1 and att B2 reaction sites. The lengths of the PCR products ser-5 , ser-3 , tph-1 and tbh-1a are 1,848, 2,230, 2,420 and 1,758 bp, respectively. The BP reaction sites att B1 and att B2 were inserted into the initiation and terminal sites of the sequences for tetanus toxin light chain ( TeTx ), R-GECO1 , Archaerhodopsin gene from Halorubrum strain TP009 ( ArchT ), TRVP1 , HisCl1 , flp-sl2-flp and GFP using PCR. These PCR fragments flanked by att B sites were recombined with the att P1 and att P2 sites in the pDONR221 vector using BP recombination reactions to generate the entry clone slot2. To generate entry clone slot3, the sl2-GFP or unc-54(3′UTR) fragments with the inserted BP reaction sites att B2r and att B3 were recombined with the att P2r and att P3 sites in the PDONR-P2R-P3 vector using the BP recombination reactions. Next, we used LR reactions to construct expression plasmids, such as the following: sra-6p::flp-sl2-flp, sra-6p::R-GECO1, gpa-4p::R-GECO1, gpa-4p::ArchT-GFP, gpa-4p::TeTx::sl2-GFP, gpa-4p::trpv1::sl2-GFP, srh-142p::trpv1::sl2-GFP, ser-5p::ser-5::sl2-GFP, tph-1p::tph-1::sl2-GFP, ceh-2p::R-GECO1, srh-142p::R-GECO1, mod-5p::R-GECO1, srh-142p::TeTx::sl2-GFP, srh-142p::ArchT-GFP, srh-142p::tph-1::sl2-GFP, ser-3p::ser-3::sl2-GFP, gpa-4p::ser-3::sl2-GFP, tbh-1p::tbh-1::sl2-GFP, tbh-1p::R-GECO1, tbh-1p::TeTx::sl2-GFP, tbh-1p::ArchT-GFP and unc-9p::GFP . To specifically express TeTx , ArchT, ser-5 , TRPV1 and HisCl1 in ASH neurons, we employed a FLP–FRT site-specific recombination system. We used fusion PCR to get a fragment of att B1:: frt-stop-frt-gene::att B2, then use BP reactions to construct slot2 donor vectors. Using LR reactions, we generated the following listed expression plasmids: gpa-11p::frt-stop-frt-TeTx::sl2-GFP , gpa-11p::frt-stop-frt-ArchT::sl2-GFP , gpa-11p::frt-stop-frt-ser-5::sl2-GFP , gpa-11p::frt-stop-frt-trpv1::sl2-GFP and gpa-11p::frt-stop-frt-HisCl1::sl2-GFP. Ultimately, the genes of TeTx , ArchT , ser-5 , TRPV1 and HisCl1 were specifically expressed in ASH neurons through the co-injection of the plasmids sra-6p::flp-sl2-flp plus gpa-11p::frt-stop-frt-TeTx::sl2-GFP , sra-6p::flp-sl2-flp plus gpa-11p::frt-stop-frt-ArchT::sl2-GFP , sra-6p::flp-sl2-flp plus gpa-11p::frt-stop-frt-ser-5::sl2-GFP , sra-6p::flp-sl2-flp plus gpa-11p::frt-stop-frt-TRPV1::sl2-GFP and sra-6p::flp-sl2-flp plus gpa-11p::frt-stop-frt-HisCl1::sl2-GFP , respectively. Confocal fluorescence imaging All confocal fluorescence imaging was performed using an Andor (Andor Technology plc., Springvale Business Park, Belfast, UK) Revolution XD laser confocal microscope system based on a spinning-disk confocal scanning head CSU-X1 (Yokogawa Electric Corporation, Musashino-shi, Tokyo, Japan), under the control of the Andor IQ 1.91 software. The confocal system was constructed on an Olympus IX-71 inverted microscope (Olympus, Tokyo, Japan). All fluorescent images were imaged by a × 60 objective lens (numerical aperture=1.45, Olympus) and captured by an Andor iXon EM + DU-897D EMCCD camera. The images were displayed and analysed using Image J 1.43b software (Wayne Rasband, National Institutes of Health, USA). Behavioural assays All the behavioural experiments were performed with young adult animals maintained at 20 °C. The assay plates (3.5 cm nematode growth medium plates (NGM)) were prepared daily. CuSO 4 was dissolved in M13 buffer consisting of 30 mM Tris, 100 mM NaCl and 10 mM KCl. To examine a single worm response to Cu 2+ stimulation, the ‘dry drop test’ was used [25] . Briefly, a micro-drop (approximately a few hundreds of nanolitres) of Cu 2+ solution was delivered via a glass micropipette in front of an animal exhibiting forward sinusoidal locomotion, and the rapid backward movement was observed and recorded when the animals encountered the repellent, of which the solution drop had been absorbed into the agar, under a Zeiss Discovery V8 stereomicroscope (Carl Zeiss MicroImaging GmbH, Göttingen, Germany). The image sequences were captured with an Andor iXon EM + DV885K EMCCD camera. To compare the data from different animals, the quantitative analysis of the behavioural parameters was performed using a custom-written script in MATLAB (Mathworks, Inc., Natick, MA) software. The duration of the reversal was calculated as the time between the initial head reversal and when the tail ceased backward movement. The body bend was defined as the change in the direction of propagation of the part corresponding to the posterior bulb of the pharynx along the y axis of the worm, assuming the worm was travelling along the x axis. NC was used to quantify the undulatory kinematics of the reversal over time [25] , [26] . First, the total length of the worm body from head to tail (head=0; tail=1) was divided into ten equal segments. Next, the midline of the animal was extracted and divided into 21 equally spaced points from head to tail. The NC of each part of the worm body was subsequently defined by the NC of each even number of points. The mean of absolute value of the NC during a reversal was defined as the magnitude of the NC, corresponding to the bending magnitude. For testing 5-HT and neuron-specific capsaicin activation in the dry drop test, 5-HT (final concentration 5 mM) and capsaicin (final concentration 10 μM) were added to liquid NGM just before pouring to prepare the assay plates. The worms were allowed to rest and adapt to the assay plates for 10–15 min before starting the test. To examine a mass animal response to CuSO 4 stimulus, we used the quadrant assay with some modifications [27] . The worms were washed four times with M13 buffer and placed on the centre of the quadrant assay plates (9 cm NGM plates) ( Fig. 1b ), which was partitioned into four regions with or without 10 mM CuSO 4 . For the exogenous capsaicin and 5-HT quadrant assay, the four regions in the tested plate were filled with capsaicin (final concentration 10 μM) and 5-HT (final concentration 5 mM), respectively, which were added into the agar media just before pouring. After 30 min, the numbers of worms over the repellent and control areas were counted. The avoidance index was calculated as (A−B)/(A+B) shown in Fig. 1b , where A is the number of worms over the repellent area and B is the number of worms over the control area. Calcium imaging Neuronal calcium responses in the soma were measured by detecting changes in the fluorescence intensity of R-GECO1, a sensitive, rapid kinetic calcium indicator of weak photobleaching [31] . A home-made microfluidic device was used for calcium imaging as previously described [32] , [33] . Briefly, a young adult animal was transferred from food to M13 buffer solution to wash food off the body. For exogenous histamine calcium imaging, the worm was transferred from food and starved for 30 min in M13 buffer or M13-histamine solution (final concentration 30 mM) [43] . Then, the worm was loaded into a home-made microfluidic device with its nose exposed to buffer under laminar flow. Stimuli were delivered in M13 buffer with or without CuSO 4 (final concentration 10 mM), capsaicin solution (final concentration 100 μM), CuSO 4 plus capsaicin and histamine (final concentration 30 mM), using a programmable automatic drug-feeding equipment (MPS-2, InBio Life Science Instrument Co. Ltd, Wuhan, China). R-GECO1 was excited by 525–530 nm light emitted by an Osram Diamond Dragon LTW5AP light-emitting diode (LED) model (Osram, Marcel-Breuer-Strasse 6, Munich, Germany) constructed in a multi-LED light source (MLS102, InBio Life Science Instrument Co. Ltd) and filtered with a Semrock FF01-593/40-25 emission filter (Semrock, Inc., NY, USA), under an Olympus IX-70 inverted microscope (Olympus) equipped with a × 40 objective lens (numerical aperture=1.3, Zeiss, Germany). Fluorescence images were captured with an Andor iXon EM + DU885K EMCCD camera with a 100-ms exposure time and 256 × 256 pixels at ten frames per second. The imaging sequences were subsequently analysed using custom-written MATLAB scripts. For Ca 2+ fluorescence imaging in ASHs, the neurons were exposed under fluorescent excitation light for 1–2 min before recording, to eliminate the light-evoked calcium transients. Each animal was imaged once. The average fluorescence intensity within the initial 5 s before stimulation was taken as basal signal F 0 . The per cent changes in fluorescence intensity relative to the initial intensity F 0 , Δ F =( F – F 0 )/ F 0 × 100%, were plotted as a function of time for all curves. The mean values of Ca 2+ signals and s.e.m. were plotted in various colours as indicated and in light grey, respectively, using IGOR Pro 6.10 (Wavemetrics, Portland, OR, USA). ‘On’ and ‘Off’ indicate Ca 2+ signals to the presentation and removal of Cu 2+ stimulation, respectively. For statistical analysis of the on and off responses, the Δ F and F 0 for the on-response are defined as the fluorescence changes during the application of CuSO 4 and the average fluorescence intensity of 5 s before the Cu 2+ stimulation, and the Δ F and F 0 for off-response are defined as the initial fluorescence changes 5 s after the removal of CuSO 4 and the average fluorescence intensity of the last 5 s of the on-response, respectively. The delay time was calculated as the time of stimulus application to the time when the single-exponential fitted curve of individual Ca 2+ on-response trace cuts fitted straight line of basal Ca 2+ signals before stimulation. Optogenetic experiments To optogenetically inhibit the studied neurons, we used ArchT, a high light-sensitive light-driven outward proton pump, driven by neuron-specific promoters to hyperpolarize the neurons [34] . Worm strains expressing ArchT were raised on 3.5 cm NGM plates seeded with Escherichia coli OP50 and All-Trans-Retinal (Sigma, final concentration of 500 μM) or without All-Trans-Retinal as a control. Animals were maintained in the dark unless otherwise indicated. ArchT was excited by 525–530 nm green light emitted by an Osram Diamond Dragon LTW5AP LED model, with adjustable intensity constructed in the MLS102 multi-LED light source. Statistical data analysis All statistical analysis was performed using SPSS software V19.0 (IBM, Armonk, NY, USA). We used one-way analysis of variance to test the means among three or more than three samples, and used two-way analysis of variance to determine the significant difference between groups for two factors (that is, the first factor was segment of body, the second factor was strains). Next, we used Bonferroni t -test correction for multiple comparisons. The results are presented as the mean values±s.e.m., with the number of experimental replications ( n ). Asterisks denote the statistical significance compared with the control: *** P ≤0.001; ** P ≤0.01; * P ≤0.05. How to cite this article : Guo, M. et al. Reciprocal inhibition between sensory ASH and ASI neurons modulates nociception and avoidance in Caenorhabditis elegans . Nat. Commun. 6:5655 doi: 10.1038/ncomms6655 (2015).